Copper nanoparticle heterogeneous catalytic ‘click’ cycloaddition confirmed by single-molecule spectroscopy Colloidal or heterogeneous nanocatalysts can improve the range and diversity of Cu(I)-catalysed click reactions and facilitate catalyst separation and reuse. Catalysis by metal nanoparticles raises the question as to whether heterogeneous catalysts may cause homogeneous catalysis through metal ion leaching, since the catalytic process could be mediated by the particle, or by metal ions released from it. The question is critical as unwanted homogeneous processes could offset the benefits of heterogeneous catalysis. Here, we combine standard bench scale techniques with single-molecule spectroscopy to monitor single catalytic events in real time and demonstrate that click catalysis occurs directly at the surface of copper nanoparticles; this general approach could be implemented in other systems. We use ‘from the mole to the molecule’ to describe this emerging idea in which mole scale reactions can be optimized through an intimate understanding of the catalytic process at the single-molecule—single catalytic nanoparticle level. The Cu(I)-catalysed 1,3-dipolar Azide-Alkyne Cycloaddition (CuAAC) click reaction introduced independently by Sharpless [1] and Meldal [2] in 2002, finds utility in many disciplines beyond synthetic organic chemistry [3] , [4] , [5] , [6] , [7] . There is an interest in improving efficiency, reducing cost as well as byproducts, and discovering new catalysts [5] , [7] , [8] , [9] , [10] , [11] , [12] for this powerful conjugation tool. Copper nanoparticles (CuNP) are being explored as click catalysts in the hope of improving reusability and efficiency compared to their solution counterparts [13] , [14] , [15] , [16] , [17] , [18] , [19] , [20] , [21] . Despite recent proof-of-concept examples of CuNP-catalysed click reactions, few investigate the catalytic activity of CuNP, and generally it is difficult, if not impossible, to establish if the true catalyst is the CuNP, copper ions leaching from it [22] , or if the CuNP acts as a reductant converting Cu(II) to Cu(I). The question as to whether heterogeneous catalysts promote homogeneous catalysis is as common as it is difficult to answer [23] . In a recent click study using Cu/Fe nanocatalysts, this question was examined in some detail allowing the identification of systems involving true heterogeneous catalysis, and those where catalysis was due to leaching, including extreme examples where the ‘catalyst’ dissolved in the reaction media [20] . Cases where heterogeneous catalysis prevails in spite of ion leaching, whether or not these ions are also catalysts, are difficult to characterize [24] , [25] , [26] . Single-molecule microscopy has been employed by Blum and co-workers [27] , [28] to unequivocally determine the heterogeneous versus homogeneous nature of a ruthenium polymerization catalyst, where the latter was found to dominate. While examples to determine the phase of the catalyst remain rare, discerning the active regions of catalysts has been the focus of a number of recent single-molecule catalysis reports. Hofkens and co-workers [29] , [30] utilized single-molecule techniques to map the catalytic activity of zeolites and mesoporous materials. Single-molecule techniques have also been used to observe crystal-face-dependent catalysis of layered double hydroxides [31] , and face-dependent catalysis of gold nanoparticles [32] , [33] , [34] and has also been the subject of recent reviews [35] , [36] , [37] , [38] . Chen and co-workers [39] have also taken a single-molecule approach to high-throughput catalyst screening, which uses single-molecule catalysis to identify high activity catalyst particles in mixtures of catalysts and activity correlations to assess reactions that do not involve fluorescence. In our strategy here, we apply the nascent area of single-molecule techniques to establish if catalysis is truly heterogeneous. Further, for those cases where improving the heterogeneous nature of the reaction is desirable, single-molecule–single nanoparticle studies can be a powerful tool for catalyst optimization [27] , [28] , [29] , [36] , [37] , [38] , [39] . In this study, we combine mole scale reactions with single-molecule studies utilizing total internal reflection fluorescence microscopy (TIRFM), an effective tool in studying heterogeneous nanoscale catalyst surface dynamics and reactivity [27] , [29] , [30] , [31] , [32] , [33] , [34] , [35] , [36] , [37] , [38] , [39] , [40] , [41] . The success of TIRFM as a single-molecule technique hinges on the generation of an evanescent wave at the glass-sample interface that only allows irradiation of the sample within approximately 100 nm from the glass support surface [42] . Single-molecule microscopy requires a change in optical signal in order to measure a molecular response. The preferred signalling processes are those that activate emission from a dye or shift its emission wavelength. Chemical reactions studied with single-molecule microscopy can be separated into two categories: those that change the structure of a molecule altering its emission properties [31] and those that require a tag such as an attached dye to probe the reaction [43] ; the dyes in these two categories have been termed participants and spectators, respectively [38] . The CuAAC click reaction falls into the second category since azide and alkyne reactive groups do not emit and an attached dye is required to visualize the reaction. Förster resonance energy transfer (FRET) between pairs of dyes have been extensively used as molecular rulers in TIRF microscopy (for example, to study protein–protein interactions) [44] , [45] , [46] , [47] , [48] , [49] . This strategy can be applied in the investigation of the CuAAC click reaction using heterogeneous catalysts by using appropriately functionalized azides and alkynes. We demonstrate here that CuNP can catalyse the click reaction between an alkyne conjugated to a donor dye and an azide modified with an acceptor dye; further, we show that the process involves true heterogeneous catalysis, rather than homogeneous catalysis induced by ions released from the CuNP. The product of the reaction is a 1,2,3-triazole that brings the two dyes in close proximity, thus enabling FRET energy transfer; this results in an acceptor emission that can be monitored by single-molecule spectroscopy. Bench-top CuNP-catalysed CuAAC The CuNP used for catalysis were prepared by a slightly modified method based on that reported by Khlobystov and co-workers [15] for the synthesis of CuNP encapsulated in hollow graphitized carbon nanofibres. The catalytic activity of these colloidal CuNP was verified at the bench-top scale in the reaction of azide 5 with phenylacetylene ( 4 ). It produced exclusively the 1,4-regioisomer 1,2,3-triazole product 6 in good yield ( Supplementary Methods and Fig. 1 ). 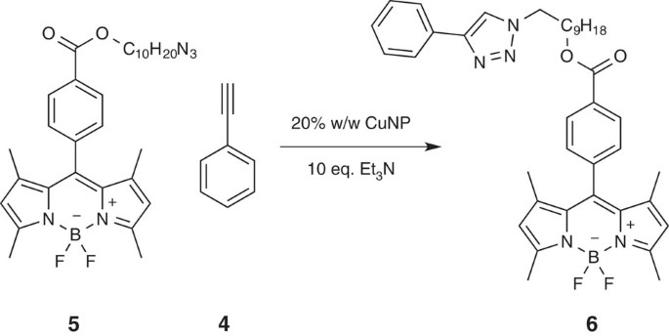Figure 1: Bench-top scale click reaction. Coupling of BODIPYazide5with phenylacetylene (4). Eq., equivalent. Figure 1: Bench-top scale click reaction. Coupling of BODIPYazide 5 with phenylacetylene ( 4 ). Eq., equivalent. Full size image Single-molecule imaging of CuNP-catalysed CuAAC For single-molecule imaging experiments, an aqueous solution of 100 pM Alexa Fluor 488 alkyne (AF488alkyne, 1 ), 100 pM Alexa Fluor 594 azide (AF594azide, 2 ) and 1 nM triethylamine was flowed at 1 ml h −1 through the flow cell reactor (Chamlide model CF-S25-B) over a round glass microscope coverslip previously spin coated with CuNP which was placed over the objective of an Olympus TIRF microscope system ( Fig. 2 , see Methods for instrument details). To image the CuAAC reaction between 1 and 2 , a solution of the two dyes was irradiated with 488 nm light and the resulting emission was recorded by an EM-CCD at 10 frames per second after being passed through a 550 long-pass filter to eliminate most of the residual donor emission. The collected emission is observed as bright bursting events on a dark background ( Supplementary Movie 1 and Fig. 2 ). 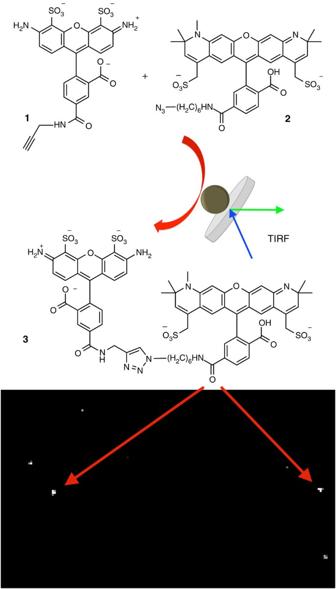Figure 2: Proposed strategy to demostrate CuNP catalysis based on FRET emission on CuAAC. CuNP-catalysed CuAAC of AF488alkyne (1) and AF594azide (2) to give click product3, and the expanded TIRFM image showing spots of AF594azide-derived emission resulting from energy transfer between 1,2,3-triazole-conjugated donor and acceptor. Figure 2: Proposed strategy to demostrate CuNP catalysis based on FRET emission on CuAAC. CuNP-catalysed CuAAC of AF488alkyne ( 1 ) and AF594azide ( 2 ) to give click product 3 , and the expanded TIRFM image showing spots of AF594azide-derived emission resulting from energy transfer between 1,2,3-triazole-conjugated donor and acceptor. Full size image The analysis of bursting at localized spots yields fluorescence intensity versus time trajectories showing stochastic intensity bursts over a dark background as shown in Fig. 3 . Still frame images time-correlated to bursting events are shown in Supplementary Fig. 1 . Sharp jumps in intensity indicate CuNP-catalysed CuAAC triazole formation creating acceptor emission from energy transferred by the excited donor. Sudden drops in intensity can be caused by a number of circumstances including fluorophore photobleaching, photoblinking or product desorption from the catalyst. 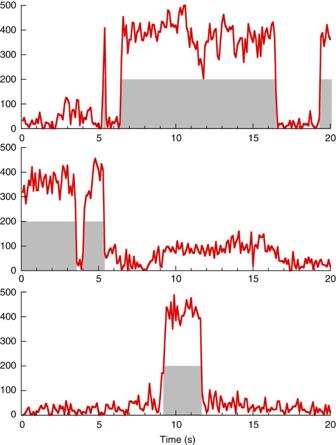Figure 3: Emission bursts of single-molecule CuAAC generated products. Representative fluorescence intensity trajectories of single catalytic spots showing multiple stochastic on/off-events. The grey areas show the times ‘on’ based on a 200-count threshold. Note that the ‘on’ times always have an intensity of about 400 counts. Figure 3: Emission bursts of single-molecule CuAAC generated products. Representative fluorescence intensity trajectories of single catalytic spots showing multiple stochastic on/off-events. The grey areas show the times ‘on’ based on a 200-count threshold. Note that the ‘on’ times always have an intensity of about 400 counts. Full size image To differentiate between dye decomposition and product desorption, we imaged a solution of 100 pM 1 , 100 pM 2 and 1 nM Et 3 N over CuNP at different laser powers. If these off-events were to be attributed to decomposition of the emissive triazole product the average ‘on’ time would be expected to be shorter with higher incident laser powers. For full laser power, the median ‘on’ time was 2.9±0.9 s (average of 26 spots) and 1.7±1.0 s for 20% power based on 47 spots ( Supplementary Figs 2 and 3 ); clearly the ‘on’ times are not longer with reduced laser power. To verify product desorption from the catalyst we synthesized 3 via classic CuAAC conditions with the in situ reduction of copper (II) sulphate and investigated its affinity for CuNP. When imaging a solution of 3 flowing over CuNP, stochastic bursting was observed throughout the focal area, which consequently disappeared when flowing water over the same catalyst. The bursting signal was subsequently recovered after flowing 3 over the catalyst again ( Supplementary Fig. 4 ). To confirm that the observed bursting is in fact due to the emission as a result of copper-catalysed click reaction enabling energy transfer between the alkyne and azide modified FRET pairs, a number of control experiments were performed using the same experimental conditions. No bright bursting spots were observed in the absence of CuNP, or when solutions containing only one or neither of the FRET pair dyes were used ( Supplementary Figs 5–8 ). The slow frame rate we used for imaging the CuNP-catalysed CuAAC of 1 and 2 leaves open the possibility that rapid diffusion of product molecules prevents us from detecting catalysis occurring in solution by Cu leached from the heterogeneous CuNP. In addressing the likelihood of this scenario, we investigated the detection limit of 3 on our instrument by imaging product 3 in solution without CuNP at 100, 10 and 1 pM. The resulting videos are represented graphically in Supplementary Fig. 9 . On our instrument, 10 pM is easily detectable; however, 1 pM is barely detectable to the trained eye; therefore, we believe that our realistic detection limit for 3 is approximately 5 pM. To clearly demonstrate catalysis occurring in the heterogeneous state on the surface of a nanoparticle requires identifying the adsorption of reagents in the same location as product generation is detected. To this end, a solution of alkyne 1 was first imaged with a 525/45 nm bandpass emission filter to observe donor emission exclusively. The emission filter was then changed to a 550 long-pass filter without moving the catalyst and a solution containing both 1 and 2 was imaged with the same 488 nm incident irradiation. 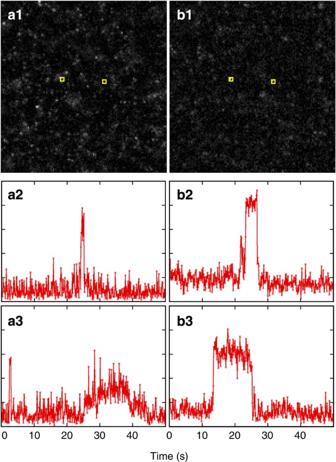Figure 4: Correlating alkyne coordination and product generation at the same location. TIRFM images of (a1) emission from donor (1) imaged with 525/45 nm bandpass filter and (b1) acceptor-derived emission resulting from energy transfer between 1,2,3-triazole-conjugated donor and acceptor imaged with a 550-nm long-pass filter. Yellow boxes highlight identical locations in the two images from which the corresponding fluorescence intensity trajectories (a2,3andb2,3) of single catalytic spots showing stochastic on/off-events were derived. The trajectories show that bursting resulting from donor emission (a2,a3) occurs in the same location as bursting originating from the triazole-forming CuAAC reaction-enabled FRET activation of acceptor (b2andb3). Figure 4 a1 , b1 represents still frame images from these experiments with yellow boxes highlighting two regions that are in identical locations in each image. These regions are examples of the alkyne coordinating to a CuNP imaged using the 525 BP filter, and subsequent CuAAC of 1 and 2 is imaged with the 550 LP filter in the same location. Discrete bursting events in these locations are visualized with the intensity versus time trajectories of these regions ( Fig. 4 a2 , 3 and b2 , 3 ). Figure 4: Correlating alkyne coordination and product generation at the same location. TIRFM images of ( a1 ) emission from donor ( 1 ) imaged with 525/45 nm bandpass filter and ( b1 ) acceptor-derived emission resulting from energy transfer between 1,2,3-triazole-conjugated donor and acceptor imaged with a 550-nm long-pass filter. Yellow boxes highlight identical locations in the two images from which the corresponding fluorescence intensity trajectories ( a2 , 3 and b2 , 3 ) of single catalytic spots showing stochastic on/off-events were derived. The trajectories show that bursting resulting from donor emission ( a2 , a3 ) occurs in the same location as bursting originating from the triazole-forming CuAAC reaction-enabled FRET activation of acceptor ( b2 and b3 ). Full size image Single-molecule emission spectra Employing the Andor spectrograph equipped on our single-molecule microscope system, we measured the emission spectra of bright events observed when a solution of 100 pM donor 1 , 100 pM acceptor 2 and 1 nM Et 3 N was flowed over CuNP. With 488 nm excitation, the emission spectra of bursts exhibit two different peaks, one centred around 520 nm and the other around 615 nm, corresponding to 1 and 2 respectively ( Supplementary Fig. 10 ). The two traces in Fig. 5 display very different relative intensities of the 520 and 615 nm emissions. The blue trace is dominated by an emission corresponding to 1 with emission from 2 appearing as a small shoulder; while the band from 2 is much more intense in the red trace. 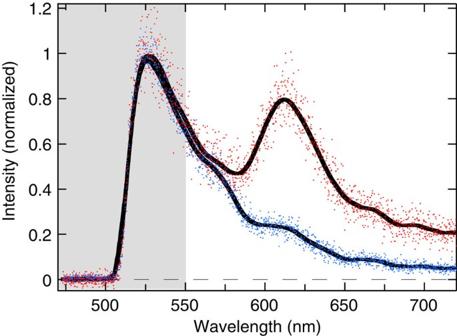Figure 5: Single-molecule emission spectra. Emission spectra (blue and red points) of two different bright spots and the spectral region excluded in TIRFM experiments by a 550 LP filter (grey area). The spectra show the emission of both1and2, indicating that CuNP-catalysed CuAAC has occurred enabling energy transfer from chromophore1to2. Figure 5: Single-molecule emission spectra. Emission spectra (blue and red points) of two different bright spots and the spectral region excluded in TIRFM experiments by a 550 LP filter (grey area). The spectra show the emission of both 1 and 2 , indicating that CuNP-catalysed CuAAC has occurred enabling energy transfer from chromophore 1 to 2 . Full size image Alkyne concentration effect Videos showing bursting events as they occur at full laser power with concentrations of 1 of 300 and 100 pM were recorded (the 100 pM video is available as a Supplementary Movie ). 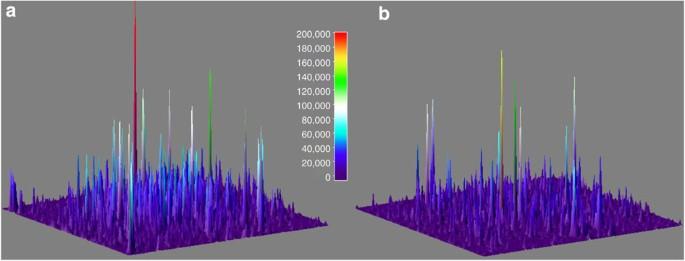Figure 6: Effect of alkyne (1) concentration. 3D-accumulated bright events (500 frames) at1concentration of 300 pM (a) or 100 pM (b), both with 100 pM2and 1 nM Et3N. The area shown corresponds to an 80-μm square. Figure 6 depicts an attempt to show the effect in a printable graph. A three-dimensional (3D) surface projection of this experiment repeated at 3 × the concentration of alkyne (300 and 100 pM 1 , 100 pM 2 and 1 nM Et 3 N) highlights the availability of open active sites on the catalyst manifested through a marked increase in product-forming events in the same time frame ( Fig. 6 ). Figure 6: Effect of alkyne ( 1 ) concentration. 3D-accumulated bright events (500 frames) at 1 concentration of 300 pM ( a ) or 100 pM ( b ), both with 100 pM 2 and 1 nM Et 3 N. The area shown corresponds to an 80-μm square. Full size image CuAAC with supported CuNP The catalytic properties of CuNP were established in a system involving supported nanoparticles. For this purpose, we chose the mesoporous silica MCM-41 as support and the two BODIPY dyes ( 5 and 7 ) with identical chromophores that differentiate only at the terminal end of a tethered carbon chain, one with an alkyne group, the other an azide ( Fig. 7 , see Supplementary Fig. 11 for spectral properties). 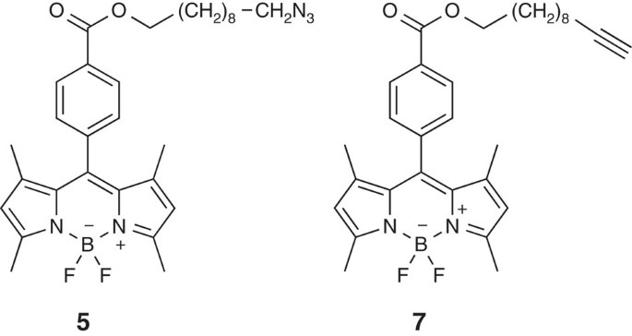Figure 7: Azide and alkyne modified BODIPY probes. Structures of BODIPY dyes5and7. Figure 7: Azide and alkyne modified BODIPY probes. Structures of BODIPY dyes 5 and 7 . Full size image When a 1 nM solution of the alkyne 7 was flowed over CuNP@MCM-41 and irradiated with 488 nm light, emissive bursts were observed that effectively mapped the MCM-41 particle ( Supplementary Figs 12 and 13 ). Conversely, when the same experiment was repeated with a solution of azide 5 , no emissive bursts were observed ( Supplementary Fig. 14 ). For our work, Alexafluor 488 alkyne (AF488alkyne, 1 ) and Alexafluor 594 azide (AF594azide, 2 ) dyes ( Fig. 2 ) were chosen as FRET donor/acceptor pair, since they exhibit good photostability, excellent FRET overlap and optimal spectral properties for 488 nm laser irradiation [47] . AF488alkyne has large absorption at 488 nm, while AF594azide absorbs very little at 488 nm ( Supplementary Fig. 10 ) maximizing FRET efficiency between the donor and acceptor and diminishing the effect of direct acceptor excitation. In single-molecule studies, concentrations in the picomolar range help make the effect of non-specific energy transfer statistically negligible [49] . Copper-catalysed cycloaddition between 1 and 2 brings the donor and acceptor close to each other allowing the AF594 acceptor to emit light following energy transfer from a proximal excited AF488 (see structure 3 ). Although CuNP-catalysed CuAAC have been shown to proceed with good efficiency [13] , it is often the case that the rate of reaction suffers dramatically at low reactant concentrations. To overcome this issue, amines such as triethylamine are commonly added in CuAAC chemistry as ligands to accelerate the reaction and protect the catalyst by facilitating coordination of the azide to copper and preventing the formation of unreactive polynuclear copper(I) acetylides [3] . Numerous bright emitting spots are observed in the resulting captured microscope video (video included as Supplementary Movie ); the trajectories for 3 show the bursting emission of single catalytic spots. The bursting reveals that the catalytic spots repeat themselves, ruling out random solution events. On average, these spots are ‘on’ about 30% of the time with ‘on’ events lasting an average of ~3 s. Time-correlated still frame images of a single bursting spot are shown in Supplementary Fig. 1 . Although unlikely at picomolar concentration, considering a resolution of a few hundred nanometres, each bright spot could potentially contain multiple donor and acceptor pairs of molecules. Analysing the intensity of bursting bright spots provides information on the number of emitters within a bright spot. The rise and fall of intensity level in the trajectories in Fig. 3 is consistent with bursts where the bright spot is due only to a single donor and acceptor pair. Multiple dyes within a bright spot often result in a step-wise change in ‘on’ intensity within a trajectory [32] . Each on–off event in the trajectory represents one catalytic turnover, where a sharp jump in intensity from the baseline denotes a catalytic product-forming event, and a sudden drop in intensity marks product degradation or desorption from the catalyst; power dependence studies support the latter. Thus, to establish if ‘off’ events resulted from product migration away from the catalytic site or were due to photobleaching, we compared the ‘on’ time of bursts at different laser powers; increased power should reduce the duration of ‘on’ events if off-events were due to photobleaching (that is, photodegradation of 3 ). The determined median ‘on’ time indicates that ‘off’ events are not the result of photobleaching, and thus can be attributed to photophysical blinking or, more plausibly, migration away from the evanescent field region. The disappearance of signal when flowing water after 3 ( Supplementary Fig. 4 ) suggests the triazole product does not have such a strong affinity for CuNP and ‘off’ events can thus be attributed to product migration out of the evanescent field. Although 3 contains many functional groups that may chelate to Cu, this result is not unexpected since the surface of CuNP is modified with alkylthiolates preventing low-affinity binding. Since emission bright spots are repeated at a single location and the reagents are being flowed over the catalyst, a nanoparticle must be at this location catalysing the reaction; thus, localized bursting behaviour is clearly indicative of nanoparticle catalysis, as catalysis due to leaching would be expected to occur at random locations. Despite proof that triazole 3 has no strong affinity for CuNP ( Supplementary Fig. 4 ), one can argue that Cu (I) ions leached into solution are homogeneously catalysing CuAAC, and that the slow imaging frame rate prevents us from observing FRET enabled emission from 3 until it binds to heterogeneous CuNP. Nevertheless, based on the measured detection limit of our instrument, 5 pM of CuAAC product 3 or 5% of the theoretical yield would have originated from homogeneous catalysis in order to meaningfully contribute to the detected signal. At realistically less than quantitative conversions, the contribution of homogenous catalysis would need to substantially increase in order to be observable. While this does not exclude the possibility of homogeneous catalysis, it strongly solidifies our conclusion favoring heterogeneous catalysis. A unique benefit of the flow reactor microscopy cell in which we perform TIRF imaging is the ability to seamlessly change the reagent solution without disturbing the microscope optics or displacing the sample, allowing us to image the same catalyst particles under various experimental conditions. Figure 4 shows still frames from experiments imaging alkyne 1 with a 525/45 nm BP filter followed by imaging a solution of 1 and 2 with a 550 LP filter showing two highlighted regions that are in the exact location in each experiment. The trajectories provided show the mean intensity of these 3 × 3 pixel areas monitored over time for each of these two locations in both experiments; they clearly demonstrate that stochastic bursting from the donor is observed in the same location as bursting from the acceptor via FRET solidifying our conclusion of heterogeneous over homogeneous catalysis. We were also able to measure the emission spectra of multiple bright emitting spots within a single focal area using an Andor spectrograph coupled to our inverted microscope fluorescence lifetime imaging microscope (FLIM)/TIRF system. AF594azide absorbs very little 488 nm light; therefore emission from direct excitation is not anticipated. Rather, the observed emission at 615 nm is due to AF594 emission from an excited state generated by energy accepted from an excited donor molecule. The difference in these two spectra in Fig. 5 is likely attributed to partial quenching of acceptor emission in the blue trace leaving donor emission [47] , [50] . These spectra ( Fig. 5 ) were measured without any emission filter allowing the entire spectrum to be collected, but in TIRF experiments, any residual donor emission that is not removed by the 550 nm long-pass filter is not resolved into discreet bursting events, but rather results in non-specific emission that contributes to the background signal (See Supplementary Fig. 15 ). This verifies the bursting observed in TIRFM experiments is due to CuNP-catalysed CuAAC linking FRET pairs, enabling energy transfer from donor to acceptor. We also looked at the effect of the concentration of 1 on the catalytic events in order to address three questions: (a) Are the catalyst active sites saturated at 100 pM 1 ? ; (b) Is the frequency of ‘on’ events affected by the concentration of 1 ? and (c) Can 1 displace product 3 from the catalytic sites? We note that positive answers to questions (b) and (c) would result in faster catalysis in ensemble experiments; single-molecule experiments can address both questions independently. As the amount of catalyst was maintained, an increasing number of bursts and their intensity with higher concentration of alkyne signifies that the catalyst active sites are not saturated at 100 pM 1 and multiple alkyne molecules can coordinate to CuNP resulting in faster catalytic turnover ( Fig. 6 ). As already noted, higher concentrations of 1 lead to increased frequency of catalytic events, indicating that at the lower concentration (100 pM 1 ), the catalytic sites are not saturated with 1 , and thus more sites are activated as the concentration of 1 increases. We expected that 1 would contribute to the displacement of the reaction product 3 because this phenomenon has been previously observed in the catalytic reduction of rezasurin on gold nanoparticle [32] , [33] , [36] . When the concentration of 1 was increased from 100 to 300 pM, however, an increase was not observed within the error of the measurement: 2.9±0.9 s at 100 pM and 1.8±1.5 s at 300 pM both based on 26 randomly selected spots ( Supplementary Figs 2 and 16 respectively). The absence of detection of a change in displacement rate may be due to the current limitations of single-molecule approaches to detect small changes or due to the limited working concentrations associated with these experiments, or may reflect that the concentration of 1 has no effect on the displacement rate under the conditions of our experiment. The concentration effect observed in Fig. 6 would be expected to be more important at typical organic synthesis concentrations (as much as 10 6 times higher than those for single-molecule work) when catalytic sites may saturate. While colloidal catalysts offer an excellent tool for mechanistic study using single-molecule techniques, in reality, they do not enable the easy catalyst separation that is usually anticipated in heterogeneous systems. Thus, beyond the single-particle CuNP-catalysed CuAAC of 1 and 2 visualized through FRET activation, we tested the catalytic properties of supported CuNP. In contrast to the Alexafluor FRET pair shown above, both chromophores of 5 and 7 absorb the incident 488 nm laser irradiation, thus are always ‘on’, resulting in greater signal compared with FRET-based single-molecule experiments and reducing the effects of scattering. With CuNP on MCM-41 (CuNP@MCM-41, see Methods), we were able to visualize the support particle on the glass coverslip. As the irradiation intensity decays exponentially from the point of total internal reflectance, effectively, only the area within approximately 100 nm of the glass coverslip surface receives laser irradiation, thus any emission detected originates only from dyes on particles near the glass surface. Since emissive bursting was observed in the case of the alkyne and not the azide, this is confirmatory evidence that the alkyne coordinates to Cu on the surface of the nanoparticle in the first step of the reaction, in a similar fashion to homogeneous CuAAC catalysts. This observation also indicates that organoazide interaction with Cu–acetylide is strongly favored over the free Cu centre, in agreement with computational and experimental reports on the involvement of Cu–acetylides in click chemistry [3] , [51] , [52] . When an organoazide coordinates to a Cu–acetylide complex, the formation of the first C–N bond is driven by the synergistic electrophilic activation of the azide and nucleophilic activation of the alkyne. Therefore, by using MCM-41 as a support, the reaction can be readily mapped to the CuNP on it, suggesting that the mechanistic details observed with colloidal nanoparticles also apply to supported systems that have the advantage of practical catalyst separation after reaction. We have demonstrated the ability of CuNP to catalyse the CuAAC click reaction on scales from bench-top to single-molecule TIRFM studies involving FRET activation through formation of 1,2,3-triazoles that bring donor-acceptor dyes in close proximity. Single-molecule studies reveal that the reaction proceeds through initial formation of Cu–acetylides on the nanoparticle surface followed by azide attack. At the concentrations used, only one catalytic event per nanoparticle takes place at a given time and the product has a residence time around 3 s following surface reaction. The systematic repetition of bursting locations is unequivocal proof that the reaction involves the CuNP surface and not ions leaching from the nanoparticle. The generic versatility of our strategy, together with studies that combine molar and molecular scales, can provide unequivocal answers as to whether a given heterogeneous catalyst operates by true heterogeneous catalysis or by promoting homogeneous catalytic events. The details of the synthesis of compounds 5 , 7 and their precursors as well as other methodological information are reported in the Supplementary Methods . The corresponding 1 H and 13 C NMR spectra for these compounds are provided in Supplementary Figs 17–23 . Transmission electron microscopy imaging and size histogram of CuNP are provided in Supplementary Figs 24 and 25 . FLIM-TIRF microscope instrumentation Fluorescence imaging was performed with an Olympus FV1000 TIRF. The instrument is equipped with a CW laser (488 nm Ar laser) and an EM-CCD (Rolera EM-C 2 , Q-Capture). The laser beam was collimated and focused through a fibre-coupling unit. A beam splitter cube with a 550-nm long-pass emission filter or 45 nm bandpass filter centred at 525 (Semrock) was used to reflect the excitation light into the oil-immersion TIR (total internal reflection) objective ( × 100, NA1.45, Olympus, PLAPO). Fluorescence spectra were recorded with a Fluorescent Lifetime Imaging System (FLIM, Microtime 200, PicoQuant). The instrument is equipped with a picosecond pulsed diode laser (485 nm, 100 ps, 40 MHz, LDH-D-C-485, PicoQuant). The laser beam was collimated and focused through a fibre-coupling unit. A beam splitter (500dcxr, Chroma) was used to reflect the excitation light into the oil-immersion TIR objective ( × 100, NA1.45, Olympus, PLAPO). The epi-fluorescent signal is passed through a 510 nm long-pass filter (Chroma) and was collected by a Spectrograph (Shamrock 163, Andor). All fluorescence microscope images were analysed using Image J (NIH). Background subtraction was performed with a rolling ball algorithm and intensity-time trajectories of bursting spots were constructed by measuring the mean intensity of 4 × 4 pixel areas for each frame. 3D surface projections of TIRF videos were done by first creating intensity sum projections and s.d. projections of the entire image stack, followed by merging of the resultant images and plotting the composite image as a 3D surface. The intensity sum projection is a simple sum of the intensity of each pixel over time, while calculating the s.d. of each pixel’s intensity value through time creates the standard deviation projection. Plotting the simple intensity sum projection on a 3D surface exaggerates long ‘on’ events, while merging the sum and s.d. projections allows for adequate representation of both long- and short-lived bursts. TIRFM sample preparation Glass coverslips (25 mm, Fisher) were cleaned by soaking in piranha solution for 30 min followed by thorough washing with MilliQ H 2 O, then dried with argon and baked at 120 °C for 5 min. The clean, dry coverslips were then placed in a solution (4% in toluene) of 3-aminopropyltriethoxysilane (APTES) and agitated on an orbit shaker (Lab-line Instruments) for 90 min, followed by successive washing with toluene, acetone, ethanol and MilliQ water. APTES treated coverslips were stored in MilliQ water until use. CuNP were deposited onto argon dried, APTES treated coverslips by spin coating 100 μl of a 0.25 mg ml −1 CuNP solution in dichloromethane at 1,200 r.p.m. The supported copper catalyst CuNP@MCM-41 was prepared by stirring a solution of CuNP (1 mg, 30% w/w) in CH 2 Cl 2 with MCM-41 for 2 h before precipitation by centrifugation at 3,500 r.p.m. and washed successively with CH 2 Cl 2 and EtOH. The product was collected by centrifugation and dried under vacuum in a desiccator. Microscopy samples for experiments using CuNP@MCM-41 were prepared by spin coating 50 μl of a suspension of the supported catalyst in EtOH (1 mg ml −1 ) onto piranha cleaned glass coverslips at 1,200 r.p.m. How to cite this article: Decan, M. R. et al. Copper nanoparticle heterogeneous catalytic ‘click’ cycloaddition confirmed by single-molecule spectroscopy. Nat. Commun. 5:4612 doi: 10.1038/ncomms5612 (2014).